Ultrafast optical tuning of ferromagnetism via the carrier density Interest in manipulating the magnetic order by ultrashort laser pulses has thrived since it was observed that such pulses can be used to alter the magnetization on a sub-picosecond timescale. Usually this involves demagnetization by laser heating or, in rare cases, a transient increase of magnetization. Here we demonstrate a mechanism that allows the magnetic order of a material to be enhanced or attenuated at will. This is possible in systems simultaneously possessing a low, tunable density of conduction band carriers and a high density of magnetic moments. In such systems, the thermalization time can be set such that adiabatic processes dominate the photoinduced change of the magnetic order—the three-temperature model for interacting thermalized electron, spin and lattice reservoirs is bypassed. In ferromagnetic Eu 1− x Gd x O, we thereby demonstrate the strengthening as well as the weakening of the magnetic order by ~10% and within ≤3 ps by optically controlling the magnetic exchange interaction. The demand for increasing density and speed in magnetic information storage has triggered an intense search for ways to control the magnetic moment by means other than magnetic fields. Following the pioneering demonstration of light-induced magnetization change on the sub-ps timescale [1] , the manipulation and control of magnetic order by ultrashort laser pulses has evolved into an exciting research topic [2] , [3] , [4] , [5] , [6] . Most of the time-resolved investigations are focused on ultrafast demagnetization [1] , [7] , [8] , [9] . This involves the quenching of magnetic order and is often described by a three-temperature model (3TM), where the coupled electron, spin and lattice subsystems are each assumed to be in equilibrium at their respective temperatures [1] , [7] . In exceptional cases, however, the photoexcitation leads to the non-thermal generation and/or enhancement of magnetic order. Enhancement is possible if the photoexcited carriers connect neighbouring magnetic sites more efficiently. For example, the ultrafast generation of ferromagnetic order in colossal magnetoresistive manganites is based on a photoactivated ‘double-exchange’ interaction between Mn 3+ and Mn 4+ ions [10] . Transient enhancement of ferromagnetism in a diluted magnetic semiconductor is mediated by photoexcited mobile carriers connecting magnetic ions (‘ p – d exchange’) [11] . These observations raise the question of whether criteria can be identified that allow us to enhance or attenuate the magnetic order of a system at will. In this article, we show that ultrafast carrier-density-controlled strengthening or quenching of the ferromagnetic order in Eu 1− x Gd x O can be achieved via resonant photoexcitation. The change of the magnetic order is established within 3 ps and detected optically via magnetization-induced second harmonic generation (MSHG). Such spin dynamics cannot be explained by a 3TM. Our theoretical analysis rather shows that the spin dynamics arises from the photoinduced non-equilibrium carrier distribution. In contrast to systems with a high carrier concentration like transition-metal, rare-earth or certain diluted-magnetic-semiconductor ferromagnets, the sub-ps carrier dynamics in low-doped Eu 1− x Gd x O is far from equilibrium due to a substantially longer electron thermalization time. The associated spin dynamics is explained by the interplay of chemically and optically generated carriers and the resulting dynamic renormalization of the RKKY-like magnetic exchange coupling. The change from ultrafast enhancement to quenching of ferromagnetism is marked by the crossover from the predominantly semiconducting to the predominantly metallic doping range of Eu 1− x Gd x O. Aside from the generalized insight into ultrafast spin as well as charge dynamics, a key requirement for spintronics technology, our investigation provides guiding information for the selection and design of materials for ultrafast optical control of magnetic order. Magnetic interaction in carrier-doped EuO Gd-doped EuO was chosen as a candidate material because of the multitude of extreme magnetism-related properties (full spin polarization, simultaneous ferromagnetic and insulator-metal transition, colossal magnetoresistance, giant magneto-optical effects and so on [12] , [13] , [14] , [15] , [16] , [17] , [18] , [19] ). Undoped EuO is a prototype Heisenberg ferromagnet. The magnetic moment of 7 μ B arises from the strongly localized, half-filled 4 f shell of the Eu 2+ ions on a cubic rock salt structure. Owing to the strong localization of the 4 f orbitals, however, the direct 4 f –4 f exchange coupling with the nearest Eu 2+ neighbours is too weak to explain the high Curie temperature of T C =69 K. Instead, the ferromagnetic order is driven by a virtual exchange mechanism [20] . Virtual magnetic excitons are created by localized 4 f electrons fluctuating into the empty Eu 5 d state so that the magnetic exchange coupling J ex can be mediated via the spatially more extended 5 d orbitals. In Eu 1− x Gd x O, J ex and T C are further enhanced by truly populating the 5 d orbitals with the extra electrons introduced by replacing Eu 2+ by the otherwise magnetically equivalent Gd 3+ , as shown in Fig. 1a [21] , [22] . Note that these dopant electrons do not form excitons, but rather occupy the Gd 5 d impurity orbitals, which in the metallic phase below T C merge with the Eu 5 d 6 s conduction band [23] to produce a long-range RKKY contribution to J ex . This mechanism raises the exciting possibility that an ultrafast enhancement of J ex may be driven by resonant optical pumping of electrons from the Eu 4 f 7 ground state to the 4 f 6 5 dt 2g magnetic exciton state ( Fig. 1b ), since this turns the virtual magnetic exciton into a real one, promoting the magnetic order. In this way, the complex, photoinduced charge dynamics results in an effective time-dependent magnetic coupling between the Eu 4 f moments. 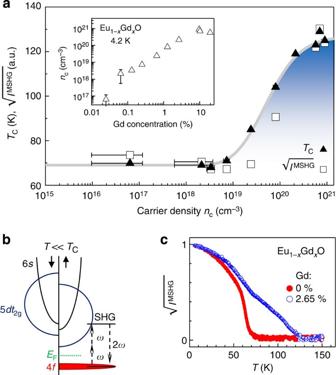Figure 1: Static magnetic properties of Eu1−xGdxO films. (a) Dependence ofTC(ref.22, solid triangles) and of the square root of the static MSHG intensity(open squares with grey line as guide to the eye) on the carrier densityncat 4.2 K in Eu1−xGdxO. The inset shows the relationship of the Gd concentration tonc(ref.22). All error bars represent the s.e.m. and the uncertainty in the film thickness in determiningncfrom the Hall measurements. (b) Sketch of the spin- and energy-dependent density of states of undoped ferromagnetic EuO near the bandgap20. The Eu 5d6sconduction band is split by the 4f–5dexchange interaction. States not shown like 4fminority, 5degand oxygen 2pare off the scale. The MSHG process probes the magnetic order via a two-photon transition to the 5d6sconduction band. (c) Temperature dependence offor undoped and 2.65% Gd-doped EuO. Figure 1: Static magnetic properties of Eu 1− x Gd x O films. ( a ) Dependence of T C (ref. 22 , solid triangles) and of the square root of the static MSHG intensity (open squares with grey line as guide to the eye) on the carrier density n c at 4.2 K in Eu 1− x Gd x O. The inset shows the relationship of the Gd concentration to n c (ref. 22 ). All error bars represent the s.e.m. and the uncertainty in the film thickness in determining n c from the Hall measurements. ( b ) Sketch of the spin- and energy-dependent density of states of undoped ferromagnetic EuO near the bandgap [20] . The Eu 5 d 6 s conduction band is split by the 4 f –5 d exchange interaction. States not shown like 4 f minority, 5 de g and oxygen 2 p are off the scale. The MSHG process probes the magnetic order via a two-photon transition to the 5 d 6 s conduction band. ( c ) Temperature dependence of for undoped and 2.65% Gd-doped EuO. Full size image Nonlinear optics probing magnetic order in Eu 1− x Gd x O An established method for probing ferroic order is SHG: emission of light at frequency 2 ω from a crystal irradiated with light at frequency ω . The susceptibility χ (2) parameterizing this conversion process is highly sensitive to the symmetry of the SHG-active compound, and since ferroic order changes the symmetry its emergence will be accompanied by the corresponding symmetry-allowed SHG components. This has been widely employed to probe the ferroic state in a multitude of oxides, including in particular the ultrafast dynamics of magnetic order [24] , [25] . In the first step, we have to scrutinize the coupling of the SHG susceptibility to the ferromagnetic order in Eu 1− x Gd x O. In general, SHG may couple to the magnetization M as order parameter or directly to the magnetic exchange interaction J ex . An expansion up to the linear terms parameterizes this: χ (2) = χ 00 + χ 10 J ex + χ 01 M + χ 11 J ex M . Here terms coupling to M (~ χ 01 , χ 11 ) are due to MSHG processes present only in the ferromagnetic phase. The other contributions (~ χ 00 , χ 10 ) do not couple to the magnetic order parameter and are therefore allowed at all temperatures. Quadratic and higher terms could be included in the expansion but, as we will soon see, they are negligible. To identify the coupling of MSHG to the magnetic order of Eu 1− x Gd x O, we performed two experiments on crystals oriented such that the crystallographic background SHG was not excited (see Methods and Supplementary Discussion on the technical details of these SHG experiments). First, in Fig. 1a , we compare the dependence of the Curie temperature T C and of the MSHG amplitude on the Gd-related carrier density n c . Here the MSHG intensity I MSHG ∝ | χ (2) | 2 was measured at 10 K, where we have a fully saturated magnetization of 7 μ B so that non-thermal changes in I MSHG at this temperature can only be related to changes in J ex . The two curves in Fig. 1a show the same qualitative dependence on n c , and the relative difference on the vertical axis never exceeds 25%. Since, according to mean-field theory, T C is proportional to J ex (ref. 23 ), we thus identify a dominating MSHG contribution coupling to J ex . Second, the temperature dependence of shown in Fig. 1c reproduces well the temperature dependence of the spontaneous magnetization M , even across the original ferromagnetic transition [22] . This includes the double-dome-like dependence in the Gd-doped samples, which is related to the complementary Eu- or Gd-driven ferromagnetic ordering processes [23] , supplemented by magnetic polaron formation [26] . Thus, these experimental results reveal a distinct dominance of the contribution from χ 11 with bilinear coupling of the MSHG amplitude to J ex and M or, expressed in terms of the measured MSHG intensity, Henceforth, we restrict ourselves to the consideration of this contribution because none of the results presented in the following are altered by this simplification. It is a particular strength of SHG that allows us to use its coupling to the ferroic state experimentally without knowing the explicit microscopy of the coupling. Because of this, the microscopy of a SHG probe signal is generally not discussed in the ‘ferroic SHG’ literature. Since, however, a coupling according to J ex M has not been discussed before, we present a possible microscopic coupling mechanism in the following. Coupling to M has been discussed a number of times in the literature [24] , [27] , [28] , [29] so that we focus on the coupling to J ex . In ref. 18 , it was shown that MSHG in Eu 1− x Gd x O is described by the equation An electric dipole (ED) and a magnetic dipole (MD) transition of the incident light field stimulate an ED emission at the doubled frequency with χ (2) as given in equation (1). When a photon is absorbed, its spin S =±1 is transferred to the system. Here an ED transition alters the orbital angular momentum, while an MD transition alters the magnetic spin of the system, according to the dipole selection rules. With only a single MD transition involved in the MSHG process in equation (2), a local spin resides in the Eu system, which must be carried away by a non-optical excitation. This occurs by coupling this local spin to the surrounding Eu spins and, hence, by generating a magnon at k ≈0 (due to momentum conservation) and, hence, ω ≈0 (the ferromagnetic magnon is a gapless excitation). The spin–spin coupling strength is parameterized by the exchange coupling constant J ex , which thus enters χ (2) . The explicit expression for this process can be derived by extending the theory for the interaction between light waves and spin waves in ref. 30 . An additional MD-type matrix element has to be added to the excitation process in ref. 30 to get from the linear optics with ED transitions to the MD-supported MSHG process in our experiment. The spin–orbit mixing contributions to the intermediately excited states in ref. 30 have to be complemented by spin–spin mixing contributions because of the involvement of the MD transition. These spin–spin exchange terms introduce the J ex dependence to χ (2) . In summary, we have introduced MSHG as a background-free probe of the magnetic order in Eu 1− x Gd x O. We have presented experimental and theoretical evidence according to which MSHG reveals the dynamics of the magnetization M and of the magnetic exchange interaction strength J ex . In Supplementary Fig. 1 and Supplementary Discussion , we discuss aspects consolidating the feasibility of MSHG for investigating Eu 1− x Gd x O magnetism in a pump/probe experiment. We show that contributions to the MSHG response that are not magnetic in origin but caused by the carrier non-equilibrium distribution after the optical excitation [31] , [32] are negligible. We also explain why crystallographic, surface and other contributions to the MSHG signal do not interfere with our experiment. 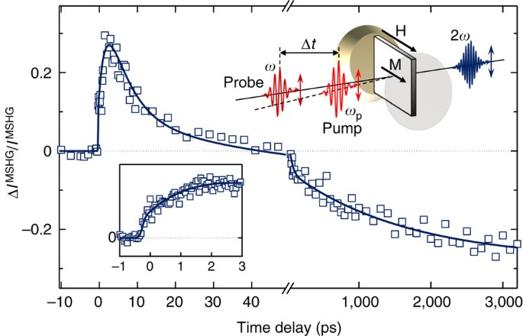Figure 2: Photoinduced spin dynamics measured by time-resolved MSHG. The time evolution of the change of the MSHG intensity at 77 K for EuO doped with 2.65% Gd is shown as a typical example. The excitation density of the pump pulse is ~380 μJ cm−2. The insets show schematics of time-resolved MSHG spectroscopy and a magnified view of the ultrafast increase of the MSHG signal. Solid lines are guides to the eye. Photoinduced spin dynamics Figure 2 shows a typical time evolution of the photoinduced change of the MSHG intensity normalized by the value before optical excitation, Δ I MSHG (Δ t )/ I MSHG (0). The data were taken at 77 K on EuO doped with 2.65% Gd. Following the photoexcitation at Δ t =0, we observe a continuous increase of the MSHG intensity up to +30% at 3 ps. This is followed by a continuous decrease passing zero at 40 ps and −25% at 3 ns. From this behaviour, we conclude that, indeed, the photoexcitation populates the 5 d orbital, resulting in an enhancement of the effective 4 f –5 d exchange J ex and, by aligning the thermally fluctuating 4 f spins, of the magnetization M . Figure 2: Photoinduced spin dynamics measured by time-resolved MSHG. The time evolution of the change of the MSHG intensity at 77 K for EuO doped with 2.65% Gd is shown as a typical example. The excitation density of the pump pulse is ~380 μJ cm −2 . The insets show schematics of time-resolved MSHG spectroscopy and a magnified view of the ultrafast increase of the MSHG signal. Solid lines are guides to the eye. Full size image The intra-atomic 4 f –5 d exchange energy of ~0.1 eV (ref. 20 ) corresponds to a time of ~40 fs so that an instantaneous MSHG increase after photoexcitation might be expected in contrast to the strikingly different time of ~3 ps. We have, however, to take into account that the magnetic exchange coupling is mediated via the RKKY interaction. The time τ 0 required to coherently establish its enhancement in the photoexcited region can be estimated from the time it takes the electronic correlation to spread through the crystal. The relevant distance is the RKKY wavelength, and the propagation velocity is the group velocity of the magnetic exciton. The latter is reduced with respect to the conduction electron group velocity by the ratio of the effective masses of the 5 d 6 s conduction electrons ( ) and of the heavy holes in the 4 f band ( ), which together form the magnetic exciton. The ratio was taken to be equal to the inverse ratio of the respective bandwidths and was extracted from literature data [23] to be ~4 × 10 3 . In addition, the low excitation energy within the conduction band of Δ E ~0.5 eV and the small wavenumber associated to this energy allows us to assume the conduction band as parabolic. Here Δ E is the difference between the pump photon energy ħω p and the 4 f –5 d 6 s gap energy E gap . With we thus obtain a build-up time τ 0 of ~8 ps, which is in reasonable agreement with the measured value of ~3 ps. The ensuing decrease of MSHG intensity on the ns timescale is associated with the demagnetization by the heating of the spin system through the transfer of the optical excitation energy from the electron system to the lattice and the spins. The observed slow relaxation is consistent with the empirical thermal demagnetization time [9] inferred from the magnetocrystalline anisotropy constant in EuO [33] , and the decrease of the MSHG intensity is consistent with the laser-pulse heating calculated from the absorption coefficient and the heat capacity of EuO [34] . Carrier-density-controlled non-equilibrium spin dynamics Investigation of the relationship between the magnetic coupling dynamics and the carrier density n c in Eu 1− x Gd x O is at the heart of our study. To simplify this investigation, the corresponding dynamics were measured at 10 K. At this temperature, the magnetic moment is fully saturated at 7 μ B per Eu 2+ ion. Hence, referring to equation (1), the non-thermal changes of the MSHG intensity are then associated to changes of J ex . 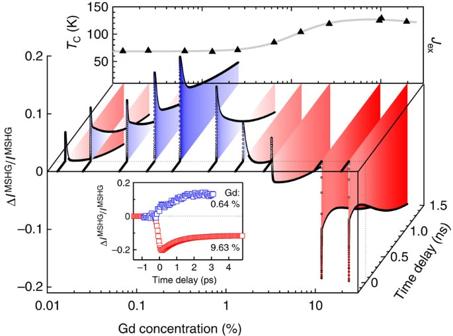Figure 3: Tuning of ultrafast spin dynamics via the control of carrier density. Change of the MSHG intensity at 10 K for Eu1−xGdxO is shown as a function of time delay and Gd concentration. For all traces the excitation density of the pump pulse is ~130 μJ cm−2, which creates a photocarrier density Δnc~1019cm−3. The inset shows a magnified view of the ultrafast change of the MSHG intensity forx=0.64% andx=9.63%. Figure 3 shows the temporal evolution of the normalized change of MSHG intensity induced by optical pumping for Gd concentrations between 0 and 19.5%. Here the laser intensity is chosen such that Δ n c ~1 × 10 19 cm −3 carriers are excited by the laser pulse. A common behaviour of all samples is the decreasing MSHG yield on a ns timescale. As mentioned above, this is caused by the thermal destabilization of the magnetic order mediated by the spin-lattice relaxation. In contrast, the MSHG response on the ps timescale depends strongly on the Gd concentration. At the lowest doping, an ultrafast increase of the MSHG signal is observed. It nicely confirms that our magneto-optical probe process reflects a variation of J ex rather than of the already saturated magnetization, in contrast to the assignment made in earlier time-resolved magneto-optical rotation measurements on undoped EuO [35] . By increasing the Gd concentration, the magnitude of this initial increase becomes progressively more pronounced and reaches a maximum near x =0.25%. Here the enhancement of the magnetic coupling exceeds an impressive 10%. (For comparison, note that the photoinduced enhancement of the p – d exchange in the diluted magnetic semiconductor systems is on the order of 0.1% (ref. 11 ).) Higher Gd doping reduces the magnitude of the initial enhancement, and at x >5% an ultrafast decrease of the MSHG signal is observed. In Fig. 4a , we summarize the pump-induced change of the MSHG yield as a function of n c at the fixed delay Δ t =3 ps. Here n c has been derived for each Gd concentration x from the relation displayed in the inset of Fig. 1a . Figure 3: Tuning of ultrafast spin dynamics via the control of carrier density. Change of the MSHG intensity at 10 K for Eu 1− x Gd x O is shown as a function of time delay and Gd concentration. For all traces the excitation density of the pump pulse is ~130 μJ cm −2 , which creates a photocarrier density Δ n c ~10 19 cm −3 . The inset shows a magnified view of the ultrafast change of the MSHG intensity for x =0.64% and x =9.63%. 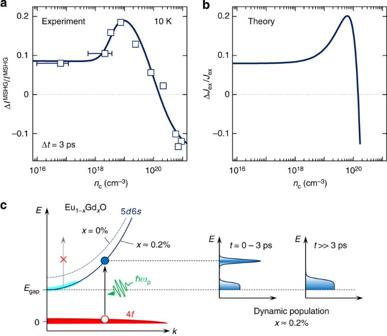Figure 4: Optical tuning of the ferromagnetic exchange interaction in experiment and theory. (a) Relation betweenncand the photoinduced change of the MSHG intensity at Δt=3 ps and at 10 K, extracted fromFig. 3. The line is a guide to the eye. Error bars forncrepresent the s.e.m. and the uncertainty in the film thickness in determiningncfrom the Hall measurements. (b) Calculated change ofJexdue to the modification of the RKKY interaction by the photoinduced non-equilibrium population of the 5d6sconduction band. Because of the expansionthe data inaare directly comparable to the theory inb. (c) Sketch of the photoexcitation dynamics beyond the 3TM in low-doped Eu1−xGdxO. The photoinduced long-lived non-equilibrium carriers modify the RKKY interaction, and thusJex. The crossed out arrow refers to photon absorption within the 5d6sconduction band, which is kinematically forbidden. For clarity, only the majority (spin-up) carriers are shown. Full size image Figure 4: Optical tuning of the ferromagnetic exchange interaction in experiment and theory. ( a ) Relation between n c and the photoinduced change of the MSHG intensity at Δ t =3 ps and at 10 K, extracted from Fig. 3 . The line is a guide to the eye. Error bars for n c represent the s.e.m. and the uncertainty in the film thickness in determining n c from the Hall measurements. ( b ) Calculated change of J ex due to the modification of the RKKY interaction by the photoinduced non-equilibrium population of the 5 d 6 s conduction band. Because of the expansion the data in a are directly comparable to the theory in b . ( c ) Sketch of the photoexcitation dynamics beyond the 3TM in low-doped Eu 1− x Gd x O. The photoinduced long-lived non-equilibrium carriers modify the RKKY interaction, and thus J ex . The crossed out arrow refers to photon absorption within the 5 d 6 s conduction band, which is kinematically forbidden. For clarity, only the majority (spin-up) carriers are shown. Full size image The growth of the MSHG response with increasing Gd concentration occurring on the ps timescale is striking. We point out that in the picture of the widely used 3TM [1] , [7] , the optical pump pulse would, in addition to exciting the localized 4 f electrons and creating the 4 f 6 5 dt 2g magnetic excitons, lead to the excitation of the chemically doped carriers in the 5 d 6 s conduction band and to their thermalization at the elevated temperature corresponding to the deposited energy. This would invariably reduce J ex since the ferromagnetic coupling with electrons in the energetically higher band states becomes weaker because of their increased wavenumber. (This behaviour of the coupling was checked by explicitly calculating the RKKY interaction for the corresponding electron distribution in the conduction band; see Supplementary Discussion .) Furthermore, the increased temperature would directly contribute to the demagnetization. Optical tuning of the magnetic coupling The key to understanding the initial increase of Δ I MSHG / I MSHG with n c in Fig. 4a is that in the low-doped Eu 1− x Gd x O the carrier thermalization time is much longer than the one in dense itinerant ferromagnets like Ni or Gd. Charge thermalization is slow because it occurs by electron–electron scattering, the rate of which is proportional to carrier concentration. In low-doped Eu 1− x Gd x O, the carrier concentration is by a factor of about 100 lower than in pure Gd. The carrier thermalization time in pure Gd equals 50−100 fs (ref. 7 ). With this the factor of 100 leads to a prolonged carrier thermalization time of low-doped Eu 1− x Gd x O of ps. We therefore conclude that the dynamics for the first few ps is dominated by a non-equilibrium charge carrier distribution, that is, the 3TM is not applicable. More importantly, since electron–electron interactions are negligible during this time period, photoexcitation of the chemically doped carriers within the 5 d 6 s band into higher band states is kinematically forbidden. Because of the large energy and the negligible momentum transferred by the photon, energy and momentum conservation cannot simultaneously be fulfilled in this two-body process. In contrast, resonant pumping of the 4 f 7 →4 f 6 5 dt 2g transition can occur because it satisfies energy and momentum conservation ( Fig. 4c ). Hence, for the first few ps after the photoexcitation, the carrier distribution is comprised of chemically doped carriers in the 5 d 6 s conduction band, which remain nearly unaffected by the pump pulse, and of the fraction of the 4 f electron population, which is photoexcited into the state with 5 d electron character. All the mobile carriers contribute to a stronger magnetic coupling between the Eu 4 f spins. This coupling mechanism is in agreement with the experimental observations on the low-doped samples but, as illustrated by Supplementary Fig. 2 , it does not explain the photoinduced attenuation of the magnetic coupling obtained when further increasing the Gd doping. For obtaining this attenuation, it is indispensable to involve an additional effect. Dynamic RKKY coupling This effect is found in the interaction between the conduction band and the Gd impurity band. An increase in the carrier density in the conduction band by chemical or photodoping strengthens its interaction with the Gd impurity band. As shown in ref. 23 , this entails an energetic downshift of the conduction band toward the Gd impurity band and, hence, a reduction of the 4 f –5 d 6 s gap energy. This shift affects the 4 f –4 f RKKY exchange. Using the many-body renormalization theory introduced in ref. 23 , we have calculated the RKKY-like coupling for the non-equilibrium electron distribution. The result is shown in Fig. 4b . In face of the crudeness of the theoretical model, the semi-quantitative, numerical agreement with the experimental result in Fig. 4a is compelling. Even without reference to the technical aspects of the calculation, which is provided as Supplementary Discussion , the non-monotonic behaviour in Fig. 4a,b can be understood, as we now describe. The density of photoexcited carriers is proportional to the spectral density at the energy ħω p − E gap addressed by the photoexcitation. Therefore, as E gap is reduced with increasing Gd doping and, thus, increasing n c , more states can be populated with photoexcited carriers (see Fig. 4c ). The enhanced density of excited carriers contributes to the increase of Δ J ex / J ex with n c . Finally, for n c >10 20 cm −3 , Δ J ex / J ex and Δ I MSHG / I MSHG get quenched for two reasons to negative values. First, with further downward shift of the conduction band the energy mismatch ħω p − E gap , and with it the wavenumber of the photoexcited carriers, increases further. Thus, because of the oscillating dependence of the RKKY coupling on the wavenumber, J ex turns over towards weaker ferromagnetic coupling. Second, with the increasingly metallic nature the electron–electron scattering time gets reduced, leading to ultrafast thermalization and concomitant magnetization quenching, that is, conventional demagnetization according to the 3TM begins to dominate. This is nicely reflected by the change of the build-up time from ~3 ps (manifestation of RKKY interaction) to ~100 fs (thermalization according to the 3TM) in the inset of Fig. 3 . In summary, we have demonstrated that the ultrafast magnetic coupling dynamics can be tuned from photoinduced enhancement to photoinduced quenching of ferromagnetic order in Eu 1− x Gd x O by controlling the carrier density. The largest enhancement of the ferromagnetic order and the crossover to quenching were observed around n c ~10 19 and ~10 20 cm −3 , respectively. This behaviour is explained by a non-equilibrium theory that extends beyond the established 3TM. It reveals that the strength of the ferromagnetic order is determined by the competing effects of the photoinduced population of the 5 d 6 s conduction band, and of the population-dependent downward shift of the conduction band. Only the combination of both effects leads to a photoinduced enhancement or attenuation of the magnetic order. Our experimental results and their theoretical modelling not only demonstrate how to control the stability of a ferromagnetic state at the ultrafast timescale, but also give a guide to the material selection and design for the dynamical optical control of magnetic order: systems with a low density of conduction band carriers (which is tuneable) but with a high density of magnetic moments (unlike, for example, in diluted magnetic semiconductors) are favourable candidates. Sample growth and characterization To study the ultrafast spin dynamics, epitaxial Eu 1− x Gd x O (001) films ( x =0−19.5%) with a thickness of 35 nm were grown under adsorption-controlled conditions on double-side-polished YAlO 3 (110) single-crystal substrates by molecular-beam epitaxy [22] . The films were protected against air by an amorphous silicon capping layer with 10–20 nm in thickness and found to be free of oxygen vacancies within the resolution limit of X-ray absorption spectroscopy [22] . Uniform growth without secondary phases was confirmed by X-ray diffraction, and the Gd concentration x was determined by prompt-gamma activation analysis and X-ray absorption spectroscopy [22] . All Eu 1− x Gd x O films possess an in-plane magnetic easy axis. Their physical properties were reported in ref. 22 . Pump-probe experiment The experimental pump-probe set-up is shown in the inset of Fig. 2 . The output of a Ti:sapphire regenerative amplifier system at 800 nm ( ħω p =1.55 eV) with a pulse width of 130 fs and a repetition rate of 1 kHz was divided into two beams. One beam was used for resonant pumping of the 4 f 7 →4 f 6 5 dt 2 g transition at 1.55 eV. The absorption length of EuO at this photon energy is about 100 nm so that the entire film was excited. The other beam was converted into a frequency-tunable beam by an optical parametric amplifier. This light was used for probing the time evolution of the ferromagnetic order by MSHG. Previous experiments revealed [18] that at 2 ħω =2.60 eV the interference by temperature-dependent linear absorption effects is avoided. We therefore chose it as the MSHG probe energy. The orientation of the sample was chosen such that crystallographic contributions to the SHG signal are suppressed so that the coupling to the magnetic order occurs free of background [18] . The MSHG yield I MSHG ∝ | P (2 ω )| 2 was measured in a normal-incidence transmission geometry under an in-plane magnetic field of 50 mT, which was applied to sustain a single-domain magnetic state. Additional technical aspects of the MSHG measurement and a discussion of its feasibility for probing the magnetization dynamics of Eu 1− x Gd x O are provided as Supplementary Fig. 1 and Supplementary Discussion . How to cite this article: Matsubara, M. et al . Ultrafast optical tuning of ferromagnetism via the carrier density. Nat. Commun. 6:6724 doi: 10.1038/ncomms7724 (2015).